High thermoelectric performance enabled by convergence of nested conduction bands in Pb7Bi4Se13with low thermal conductivity 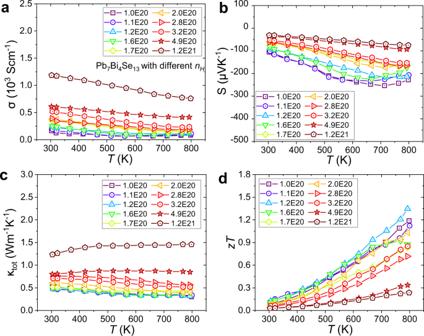Fig. 1: Thermoelectric properties. aElectrical conductivity,bSeebeck coefficient,ctotal thermal conductivity, andddimensionless figure of merit,zT. Thermoelectrics enable waste heat recovery, holding promises in relieving energy and environmental crisis. Lillianite materials have been long-term ignored due to low thermoelectric efficiency. Herein we report the discovery of superior thermoelectric performance in Pb 7 Bi 4 Se 13 based lillianites, with a peak figure of merit, zT of 1.35 at 800 K and a high average zT of 0.92 (450–800 K). A unique quality factor is established to predict and evaluate thermoelectric performances. It considers both band nonparabolicity and band gaps, commonly negligible in conventional quality factors. Such appealing performance is attributed to the convergence of effectively nested conduction bands, providing a high number of valley degeneracy, and a low thermal conductivity, stemming from large lattice anharmonicity, low-frequency localized Einstein modes and the coexistence of high-density moiré fringes and nanoscale defects. This work rekindles the vision that Pb 7 Bi 4 Se 13 based lillianites are promising candidates for highly efficient thermoelectric energy conversion. Worldwide energy and environmental crisis have an urgent requirement on clean and sustainable energy sources due to the combustion of fossil fuels. Thermoelectric (TE) semiconductors provide promising opportunities in enabling the conversion of waste heat into electrical energy, especially favorable for relieving the current dilemma [1] , [2] , [3] , [4] . The crucial issue is the relatively limited energy conversion efficiency, related to the TE figure of merit, zT = S 2 σ T /( κ e + κ L ). Here, S and σ are Seebeck coefficient and electrical conductivity; T is absolute temperature; κ e and κ L are electronic and lattice thermal conductivities, respectively. Electronically, the intertwining of S , σ , and κ e complicates efforts to optimize TE performance. With the single parabolic band assumption, the zT can be described as zT = zT ( η , B ) by the conventional quality factor analysis [5] , [6] . This description correlates zT solely with two independent physical parameters, i.e., tunable reduced Fermi level, η and quality factor, B . This B value is an effective descriptor with considering band degeneracy ( N v ), inertial effective mass ( m I * ), deformational potential ( Ξ ), and lattice thermal conductivity, according to the relationship of B ~ N v /( m I * Ξ 2 κ L ) [6] . The optimization of electrical properties and simultaneous suppression of heat transport are essential and critical for advanced TE materials. To achieve the optimal electrical properties, effective strategies on electronic band engineering are indispensable, such as electronic band convergence [7] , [8] , [9] , resonant level introduction [10] , [11] , band inversion and flattening [12] , [13] . Meanwhile, low lattice thermal conductivity is equivalently favorable. Intrinsically, the reduced heat transport requires large lattice anharmonicity [14] , [15] , complex crystal structures [16] , localized Einstein modes [17] , [18] , and suppressed transverse acoustic phonon branches [19] , [20] . Extrinsically, lattice imperfection engineering, including point defect [21] , [22] , dislocation [23] , [24] , grain boundary and interface [25] , coherent nanostructure [26] , [27] , etc., is equally prevalent to scatter all-length scale phonons and thus impede heat propagation. The alignment of multiple electronic bands and intrinsically low lattice thermal conductivity are highly beneficial for promising TE materials. Ternary heavy metal chalcogenides have emerged as potential candidates for optimal TE materials, especially the Pb N −1 Bi 2 Se N +2 lillianite homologous series [28] , [29] , [30] . These Pb N −1 Bi 2 Se N +2 homologous series comprise of NaCl-type layered modules with different edge-sharing octahedra. Historically, lillianite homologs have been overlooked due to their intrinsically inferior electrical properties. Theoretically, by systematically modulating the building blocks of (PbSe) m and (Bi 2 Se 3 ) n , intriguing electronic properties could be still anticipated. Furthermore, heavy constituent elements, complex crystal structure, and lone pair 6 s 2 electrons [31] in Pb 2+ and Bi 3+ collectively give rise to limited phonon propagation, large lattice anharmonicity, and thus low lattice thermal conductivity. However, it is still a grand challenge to discovery promising TE performance in lillianite homologs. Here, we report an unconventional TE compound, Pb 7 Bi 4 Se 13 . By a series of heterogeneous element doping (Ga, In, Ag, and I), a high maximum zT of 1.35 at 800 K and a decent average zT of 0.92 from 450 to 800 K are concurrently realized for n -type (Pb 0.95 Ga 0.05 ) 7 Bi 4 Se 13 , which becomes the highest performance realized not only in lillianites but also in a series of compounds with similar structures. This optimal TE performance electronically stems from the alignment of nested conduction bands. A distinctive quality factor is delicately set up to screen and evaluate TE performance. This developed quality factor incorporates non-parabolic bands and bipolar effect. It breaks the limitation of the conventional quality factor that uses single parabolic band assumption. By adopting this, a more promising TE performance is also accessible with enhanced quality factors. Equally significantly, the lattice thermal conductivity is exceptionally low of 0.17 W m −1 K −1 at 800 K, which originates from large lattice anharmonicity, low-frequency localized Einstein modes, and the coexistence of high-density moiré fringes and nanoscale defects, especially periodic defective stripes with high-density stacking faults and intense lattice strains. Our work demonstrates that Pb 7 Bi 4 Se 13 based lillianites hold a great potential to be efficient TEs. Importantly, this work also develops an unconventional approach to calculate quality factors, highly favorable for accelerating the screen and evaluation of advanced TE systems. TE performance Pb 7 Bi 4 Se 13 crystallizes in a monoclinic structure with the space group (No. 12) of C 2/ m [28] . This monoclinic structure consists of diverse polyhedra, including PbSe 6 , PbSe 7 , and BiSe 6 (Fig. S 1a ). The synthesis of Pb 7 Bi 4 Se 13 includes ball-milling and long-term annealing with details presented in the experimental section. A series of heterogeneous elemental doping has been carried out by introducing Ga, In, Ag, and I, according to the nominal compositions of (Pb 1− x Ga x ) 7 Bi 4 Se 13 ( x = 0, 0.02, 0.05, and 0.1), (Pb 1− x In x ) 7 Bi 4 Se 13 ( x = 0.05 and 0.1), (Pb 1− x Ag x ) 7 Bi 4 Se 13 ( x = 0.05 and 0.1) and Pb 7 Bi 4 Se 13− x I x ( x = 0.4 and 0.8). The XRD patterns of pristine and doped Pb 7 Bi 4 Se 13 are presented in Fig. S 1b . This distinct doping achieves varied electron concentrations at 300 K, ranging from 1.0 × 10 20 to 1.2 × 10 21 cm −3 . For the convenience of comparison and discussion, Pb 7 Bi 4 Se 13 with different element doping are denoted as the corresponding electron concentration ( n H ) measured at 300 K, as shown in the inset of Fig. 1 . The composition, carrier concentration, Hall mobility, and geometry density are tabulated in Table S1 . It should be noted that there exists a certain degree of anisotropy of TE properties, due to the monoclinic structure of Pb 7 Bi 4 Se 13 . The measurement geometry and TE properties parallel and perpendicular to the spark plasma sintering (SPS) directions of two different samples are presented in Fig. S 3 . In this work, only the TE properties parallel to the SPS direction is presented and discussed for convenience. It should be noted that zT value calculations are consistent from the direction of electrical conductivity, Seebeck coefficient, and thermal conductivity. For instance, (Pb 0.95 Ga 0.05 ) 7 Bi 4 Se 13 corresponds to the sample with n H of 1.2 × 10 20 cm −3 (also denoted as Ga2). As shown in Fig. 1a , the electrical conductivities, σ of Pb 7 Bi 4 Se 13 alloys with n H larger than 1.6 × 10 20 cm −3 , show a decreasing tendency with increasing temperature, which is a characteristic of degenerated semiconductors. The σ of Pb 7 Bi 4 Se 13 alloys with lower n H decreases firstly and then increases slightly with rising temperature. Specifically, σ of Pb 7 Bi 4 Se 13 with n H of 1.2 × 10 20 cm −3 decreases from 250 Scm −1 at 300 K to 104 Scm −1 at 723 K, followed by a slight increase to 119 Scm −1 at 800 K. The magnitude of Seebeck coefficient, | S |, of Pb 7 Bi 4 Se 13 with n H higher than 2.8 × 10 20 cm −3 increases monotonously with increasing temperature. And the | S | of samples with lower n H demonstrates broad extrema at high temperatures, attributed to the contribution from the minority carrier. Taking the sample with n H of 1.2 × 10 20 cm −3 as an example, the S at 300 K is −89 μVK −1 and decreases to −217 μVK −1 at 723 K and then increase to −213 μVK −1 at 800 K. According to Goldsmith–Sharp bandgap, E g = 2 e | S max | T max , the | S max | and T max are the maximum of the magnitude of Seebeck coefficient, and its corresponding temperature, respectively. The bandgap is estimated to be about 0.33 eV, close to the reported value of 0.29 eV [28] . The total thermal conductivities of Pb 7 Bi 4 Se 13 demonstrate low values at 300 K, e.g., 0.48 Wm −1 K −1 in Pb 7 Bi 4 Se 13 with n H of 1.2 × 10 20 cm −3 , which further decreases to 0.32 W m −1 K −1 at 800 K. By systematic doping, a series of zT is achieved. And the peak zT of 1.35 is obtained at 800 K for the composition of (Pb 0.95 Ga 0.05 ) 7 Bi 4 Se 13 with n H of 1.2 × 10 20 cm −3 (Fig. 1d ). It is worth noting that this is the highest zT achieved to date not only in lillianite homologous series, but also in a series of compounds with similar structures, such as Tetradymite, Pavonite, Cannizzarite, Galenobismuthite, complex rare-earth sulfides, and other structure-similar compounds. The total number of 37 different compounds was enumerated and compared in Fig. S 2 , which shows the competitive performance of Pb 7 Bi 4 Se 13 . The detailed lattice thermal conductivities and zT values of 37 distinct compounds are tabulated in Table S2 . Compared to the state-of-the-art TE materials, like PbTe [7] , SnSe [32] , GeTe [33] , [34] , and Mg 3 Sb 2 [35] , etc., this result demonstrates a great potential for realizing high TE performance in lillianite-type or similar structures. These promising high peak and average zT values enable Pb 7 Bi 4 Se 13 to be applicable for middle-temperature power generation, such as waste energy recovery, remote sensor power, and emergency power sources. Besides, it also could be employed in the marine engines of ships by utilizing waste heat from exhaust pipes. Furthermore, thermomechanical properties are also investigated in Pb 7 Bi 4 Se 13 . The compression test shows an ultimate compressive strength of 85 MPa and the strain can reach 1.2% (Fig. S 6 ). Nanoindentation investigation indicates the hardness of 2.88 ± 0.04 GPa (Fig. S 7 ). And the microstructural investigation shows no obvious precipitates and micropores in the sample after annealing under vacuum conditions for 2 weeks (Fig. S 8 ), which shows its reasonably robust thermal stability. The heating and cooling measurements is also presented in Fig. S 5 . Fig. 1: Thermoelectric properties. a Electrical conductivity, b Seebeck coefficient, c total thermal conductivity, and d dimensionless figure of merit, zT . Full size image Convergence of nested conduction bands To understand the origin of such high TE performance, we performed DFT calculations to study the electronic structure of Pb 7 Bi 4 Se 13 . 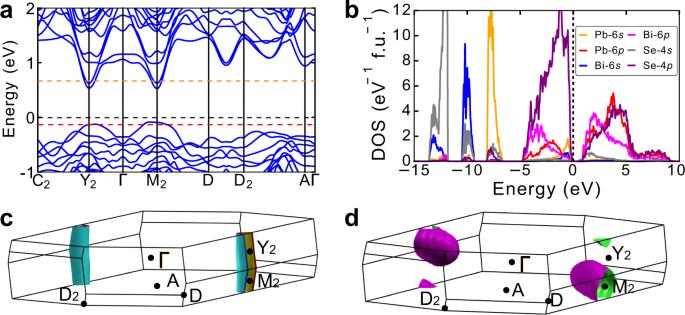Fig. 2: Electronic structure and Fermi surfaces. aBand structure. The dashed black line indicates the Fermi level of pristine Pb7Bi4Se13. The orange and red dashed lines correspond to the Fermi levels of 0.05 electron- and 0.05 hole-doped Pb7Bi4Se13, respectively.bElectronic DOS projected ontosandporbitals for each element. Fermi surfaces ofcelectron-doped Pb7Bi4Se13, anddhole-doped Pb7Bi4Se13. Figure 2a shows the band structure along with the high symmetry k -point path. The conduction bands at M 2 and Y 2 points demonstrate large E ~ k dispersion, implying the light band characteristic. The feature is the band nestification especially occurred at M 2 and Y 2 . These bands have nearly the same energies, i.e., the difference in the conduction band minimum (CBM) at M 2 point is around 100 meV, which can synergistically participate in the electrical transport. More significantly, the effectively nested conduction bands at M 2 and Y 2 also demonstrate nearly indiscernible energy separations. In details, the energy difference of CBMs of M 2 and Y 2 is as small as 8 meV. In this way, the nested conduction bands at M 2 and Y 2 reveal a high number of valley degeneracy, comparable to many decent TE materials, such as n -type Si [1] , Bi 2 Se 3 [36] , and PbTe [7] , as well as p -type elemental Te [37] . The convergence of nested bands enables multiple conducting channels without the deterioration on the Seebeck coefficient, highly favorable for superior electrical performances. A recent study suggests the convergence of electronic bands at distant k points is superior [38] . However, for semiconductors with lower symmetries, this favorable band configuration is a grand challenge. Alternatively, the convergence of nested bands could be significant to advance electrical properties for lower-symmetry TE materials. The convergence of nested bands plays an important role in charge transport properties than the situation with only heavy bands, even though it introduces a certain degree of intervalley scattering. This situation is confirmed by the theoretical calculation in the recent work [38] , in which the power factors in band configuration of nested bands are still higher than that in band configuration of the heavy band only. Experimentally, the band nestification is proven to be an advanced method in the Tellurium TE compound with space for improvement [38] . Furthermore, the convergence of nested bands holds great potential for TE materials, if nested bands could be removed away from the same k point by chemical modifications. Fig. 2: Electronic structure and Fermi surfaces. a Band structure. The dashed black line indicates the Fermi level of pristine Pb 7 Bi 4 Se 13 . The orange and red dashed lines correspond to the Fermi levels of 0.05 electron- and 0.05 hole-doped Pb 7 Bi 4 Se 13 , respectively. b Electronic DOS projected onto s and p orbitals for each element. Fermi surfaces of c electron-doped Pb 7 Bi 4 Se 13 , and d hole-doped Pb 7 Bi 4 Se 13 . Full size image In regard to valence band structure, the valence band maximum (VBM) exhibits flatten dispersion along Γ-Y 2 and Γ-M 2 -D lines, which is a characteristic of heavy valence valleys. The VBM lies in the middle of Γ-Y 2 and Γ-M 2 paths, implying high valley degeneracy. Therefore, the multiband feature in both conduction and valence valleys enables Pb 7 Bi 4 Se 13 alloys to be promising for high TE efficiency. The spin–orbital coupling (SOC) effect on the band structure is also considered. The introduction of SOC has an indiscernible effect on the band dispersions of CBM and VBM, as shown in Fig. S 9 . The calculated E g is suppressed from 0.67 eV (without SOC) to 0.22 eV (with SOC). Figure 2b exhibits the orbital projected density of states (DOS). In the region from the CBM to 1 eV above the Fermi level ( E f ), the states are dominated by p orbitals of Pb, Bi, and Se, with minor components from s orbitals of Se. The valence bands ranging from 1 eV below the E f to the VBM is dominated by Se-4 p and Pb-6 s states with minor mixed contributions of Bi-6 s , Bi-6 p , and Pb-6 p states. The 6 s 2 electrons of Pb and Bi are deeply located below Se 4 p , forming lone-pair electrons. In the band structure shown in Fig. 2a , the orange and red dashed lines represent the E f calculated from DFT for the 0.05 electron-doped and 0.05 hole-doped Pb 7 Bi 4 Se 13 . In the electron-doped Pb 7 Bi 4 Se 13 , the E f goes across two bands at both Y 2 and M 2 , which forms a nested Fermi surface consisting of two cylindrical-like electron sheets, visible in Fig. 2c . On the other hand, Fig. 2a shows that the Fermi level only lies in one band at both Y 2 and M 2 in the case of hole-doped Pb 7 Bi 4 Se 13 , and the hole pocket at M 2 is obviously larger than Y 2 , confirmed by the Fermi surface in Fig. 2d . It should be noted that nested bands could trigger strong electron–phonon scattering by the zone center phonons, which is a detrimental effect on charge transport. It is meaningful to calculate the scattering rates for each band and valley by using the electron–phonon coupling calculations based on density-functional perturbation theory, which will be the subject of our future work separately. Non-parabolic charge transport Parabolic band assumption is dominant for TE materials with wide bandgaps. For semiconductors with narrow band gaps, like PbTe [7] and CoSb 3 [8] , the non-parabolicity of electronic bands occurs, which stems from interactions between conduction and valence bands [8] , [39] . As shown in Fig. 3a , three-dimensional (3D) plots of parabolic and Kane bands are presented. The color bar is indicative of the relative energy levels. Clearly, the parabolic band reveals an ellipsoid-shaped energy surface. By contrast, the Kane band demonstrates a non-parabolic energy surface deviating from band edges. The conduction band nestification in parabolic and Kane bands are also considered. Two conduction bands are located at the same k point and flat valence bands are shown in the Brillouin zone. 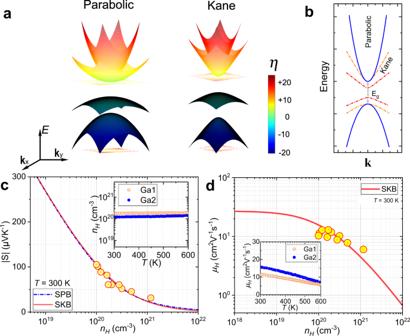Fig. 3: Electronic transport properties. a3D illustration of Parabolic and Kane bands with asymmetric conduction and valence bands. The features of conduction band nestification and relative flat valence band are presented.bE~kdispersions of parabolic (solid blue line) and Kane bands with different band gaps,Eg(orange and red dot-dash lines).cHall electron concentration,nHdependence of the magnitude of Seebeck coefficient (Pisarenko plot). The inset shows the temperature dependence ofnHof two compositions, Ga1 (red circle) and Ga2 (blue circle).dHall mobility,μHas a function ofnH. The red solid line is calculated based on the single Kane band (SKB) model. The inset shows the temperature dependence ofμHof Ga1 and Ga2. Figure 3b presents the two-dimensional (2D) dispersion relations, E ( k ) ( E energy, k wave vector). With respect to the parabolic band, E is proportional to k 2 , complying with the relationship, \(E=\frac{{\hslash }^{2}{{{{{\bf{k}}}}}}^{2}}{2{m}^{\ast }}\) . Here its effective mass, m * keeps as constant ( \({m}^{\ast }={m}_{0}^{\ast }\) effective mass at band edge). For the Kane band, it remains parabolicity at the energy extrema of electronic bands but deviates from parabolicity in a linear k tendency with departing from band edges. And the E ( k ) dispersion could be well described by \(E{{\mbox{(}}}1+\frac{E}{{E}_{g}}{{\mbox{)}}}=\frac{{\hslash }^{2}{k}^{2}}{2{m}^{\ast }}\) . Its effective mass, m * varies with Fermi level, following this relationship, \({m}^{\ast}={m}_{0}^{\ast}(1+\frac{2E}{{E}_{g}})\) [8] . Fig. 3: Electronic transport properties. a 3D illustration of Parabolic and Kane bands with asymmetric conduction and valence bands. The features of conduction band nestification and relative flat valence band are presented. b E ~ k dispersions of parabolic (solid blue line) and Kane bands with different band gaps, E g (orange and red dot-dash lines). c Hall electron concentration, n H dependence of the magnitude of Seebeck coefficient (Pisarenko plot). The inset shows the temperature dependence of n H of two compositions, Ga1 (red circle) and Ga2 (blue circle). d Hall mobility, μ H as a function of n H . The red solid line is calculated based on the single Kane band (SKB) model. The inset shows the temperature dependence of μ H of Ga1 and Ga2. Full size image To capture the effective mass of Pb 7 Bi 4 Se 13 at room temperature, the pisarenko plot based on single Kane band (SKB) and single parabolic band (SPB) assumptions could be well-simulated by the effective mass, m s * of 1.1 m e , as suggested in Fig. 3c . The temperature dependence of effective mass verifies its band nonparabolicity, as shown in Fig. S 10b . It should be noted that the Seebeck effective mass, m s * is defined as the density of state effective mass in TE community, which predicts the Seebeck coefficient with Hall carrier concentration, n H in both the SPB and SKB models. However, it should be also realized that the qualitative difference between m s * (Seebeck effective mass) and m * (effective mass from the E ~ k dispersion). The Seebeck effective mass is defined by Eqs. ( 1 ) and ( 2 ), which remain unchanged with increasing n H . Differently, the effective mass, m * defined by \({m}^{\ast }=\hslash {\left({d}^{2}E/d{k}^{2}\right)}^{-1}\) , increases with increasing E . The temperature-dependent n H of two compositions of (Pb 0.98 Ga 0.02 ) 7 Bi 4 Se 13 (Ga1, n H = 2.0 × 10 20 cm −3 ) and (Pb 0.95 Ga 0.05 ) 7 Bi 4 Se 13 (Ga2, n H = 1.2 × 10 20 cm −3 ) is presented in the inset of Fig. 3c . The n H of the two compositions remains unchanged up to 600 K. Meanwhile, the Hall mobility, μ H of all compositions as a function of n H follows the Kane-type charge transport characteristic, demonstrated by the red solid line. This n H dependent μ H considering SKB model is calculated based on the non-degenerate mobility, μ 0 at 300 K. This relationship is presented as below [40] 
    n_H=(2m_d^∗k_BT)^3/2/3π^2ℏ^3·[(2K+1)·^0F_-2^1]^2/3K(K+2)·^0F_-4^1/2,
 (1) 
    μ_H=e/√(2)m_I^∗·πℏ^4v_l^2d/Ξ^2(m_b^∗k_BT)^3/2·3K(K+2)·3^0F_-4^1/2/(2K+1)^2·^0F_-2^1,
 (2) where k B is the Boltzmann constant, ħ is the reduced Planck constant, K is the anisotropy of Fermi surface, defined by K = m ǁ */ m ⊥ *, m ǁ * and m ⊥ * exhibit the longitudinal and transverse effective mass. K is assumed to be 1 here. n F m k is the generalized Fermi integral. v l is the speed of sound, d is the sample density, m I * and m b * are inert and single-valley effective mass. Unique quality factor analysis Conventional quality factor ( B ) analysis provides an insight into TE physics. It decouples zT into the tunable reduced Fermi level, η and B , based on the SPB model (see Supplementary Note 2 ). However, this SPB model is limited to fully describe TE semiconductors with band nonparabolicity and bipolar effect [41] . At first, the discernible difference between parabolic and Kane bands, shown in Fig. 3a, b , enables non-negligible deviations by using SPB to describe the electronic transport of non-parabolic bands. Secondly, the bipolar effect frequently emerges in semiconductors with small band gaps. This effect leads to a decrease in the Seebeck coefficient and increases in thermal conductivity, which severely deteriorates TE performances at high temperatures [41] . Obviously, this bipolar effect limits the applications of conventional quality factors. Thirdly, even taking advantage of the first-principles calculation, it is still time-consuming and expensive to determinate fundamental parameters, such as effective mass, carrier relaxation time, and deformational potentials of electronic bands. Consequently, an unconventional quality factor considering both band non-parabolicity and bipolar effect is highly necessary. Herein, this unique quality factor, B * Kane is developed by using two Kane band (TKB) models. Distinct from the traditional quality factor, the zT here is closely correlated with the reduced Fermi level, η (η = (E − E f ) /k B T) , and the reduced bandgap, ξ ( ξ = E g /k B T ), which is summarized as follows 
    zT=(S_eγ +S_h)^2/(γ +1)[(k_B/e)^2γξ/3B_Kane^∗·^0F_-2^1 +(L_eγ +L_h)]+γ(S_e-S_h)^2,
 (3) And this unique quality factor B * Kane is generalized as below 
    B_Kane^∗=k_B/e^2·σ_E_0E_g/κ_L
 (4) in which the S denotes the Seebeck coefficient, L is the Lorenz number, \({\sigma }_{{{E}}_{0}}\) is the transport coefficient, γ is the electrical conductivity ratio. The subscripts, e and h , denote electrons and holes. The derivation is presented in Supplementary Note 3 . With the determination of physical parameters of the conduction band, we could obtain a series of zT values by changing B * Kane [42] . This B * Kane considers band nonparabolicity, band degeneracy N v , inertial effective mass m I * , and deformation potential Ξ . An example is provided based on Pb 7 Bi 4 Se 13 with a specific B * Kane = 6. 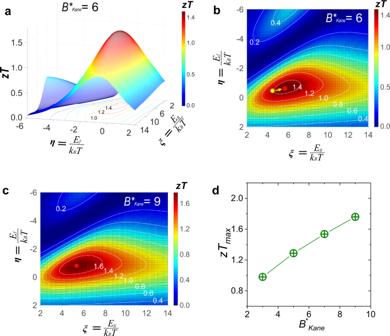Fig. 4: Quality factor analysis. a3D plot of figure of merit,zTas functions of reduced Fermi level,ηand reduced band gap, ξ.bContour plot ofη-andξ-dependentzTwith a quality factor,B*Kane= 6. The yellow dot corresponds to the experimental data of Pb7Bi4Se13withnHof 1.2 × 1020cm−3(Ga2). The red point indicates the highestzTvalue. Contour lines in white color correspond to a series ofzTvalues.cContour plot ofη-and ξ-dependentzTwithB*Kane= 9.dThe maximumzT(zTmax) as a function ofB*Kane. Figure 4a depicts the theoretical zT as functions of η and ξ . A maximum zT could be achieved with simultaneously optimized ξ and η . A contour plot is presented in Fig. 4b with the B * Kane of 6. The progressive changes in the color bar from blue to red correspond to zT from 0 to 1.48. Contour lines with representative zT values, such as 0.4, 0.8, and 1.4, are marked by dash-dot lines in Fig. 4b . Taking Pb 7 Bi 4 Se 13 with n H of 1.2 × 10 20 cm −3 as an example, its η and ξ at 800 K could be estimated to be −0.5 and 4.6, which is indicated by the yellow dot in Fig. 4b . The estimation of η , ξ , and B * Kane is presented in Supplementary Note 4 . It is worth noting that the difference in conduction and valence band is considered and included in this model by using the band anisotropy, Λ . Fig. 4: Quality factor analysis. a 3D plot of figure of merit, zT as functions of reduced Fermi level, η and reduced band gap, ξ. b Contour plot of η- and ξ -dependent zT with a quality factor, B * Kane = 6. The yellow dot corresponds to the experimental data of Pb 7 Bi 4 Se 13 with n H of 1.2 × 10 20 cm −3 (Ga2). The red point indicates the highest zT value. Contour lines in white color correspond to a series of zT values. c Contour plot of η- and ξ-dependent zT with B * Kane = 9. d The maximum zT ( zT max ) as a function of B * Kane . Full size image A maximum zT of 1.48 is predicted as represented by the red point in Fig. 4b . It can be achieved by further optimizing η and ξ, indicated by the yellow arrow. For the tuning of bandgap, the chemical substitution of selenium by sulfur or tellurium tends to enlarge and decrease band gaps, respectively. This quality factor could be further optimized via chemical modifications on electronic band structures. The introduction of coherent nanoscale defects is favorable for improving quality factors, which could guarantee unchanged carrier mobilities, concomitantly strengthen defect-phonon scattering, and further decrease lattice thermal conductivity. Specifically, this could be chemically realized by introducing nanoscale precipitates such as SrSe into Pb 7 Bi 4 Se 13 host matrix, which is proven effective in the previous work [26] . There are still a variety of effective chemical methods to increase quality factors, such as decreasing band offsets to increase effective band convergence by doping heterogeneous elements at Pb or Bi sites. If B * Kane turns into 9, the maximum zT is predicted to be 1.76 as shown by the red point of Fig. 4c . Figure 4d shows that the maximum zT is proportional to the enhanced B * Kane , which can be used as an insightful guide to exploiting high-performance TE materials. It should be noted that the quality factor with SKB model has already been established, which could evaluate and predict the TE performance [40] . However, its application is limited at low temperatures, due to thermally excited minority carriers with increasing temperatures. The contribution of minority carriers becomes inevitable and considerably deteriorates TE performances. A lack of effective quality factors brings a great challenge to evaluate and predict TE performances in semiconductors with narrow band gaps, especially at high temperatures. To resolve this issue, this unique quality factor is established with TKB model, which can provide an effective and time-saving method. The derivations on previously reported quality factors established on SPB and SKB models ( B Para and B Kane for clarity) [6] , [40] , and developed B * Kane are presented in Supplementary Note 5 . With regard to previously reported quality factors, zT values only correlate with the B Para (or B Kane ) and reduced chemical potential, η . By contrast, the zT in this unique quality factor depends on three independent variables, B * Kane , η and ξ . The 3D and contour plots of three different quality factors are presented in Fig. S 12 . This elaborately developed B * Kane not only plays a significant role in evaluating and predicting TE performance in Pb 7 Bi 4 Se 13 . It can also be extended to more TE materials with narrow bandgaps, such as prototypical (Bi,Sb) 2 Te 3 [36] and van der Waals crystal Ta 4 SiTe 4 [43] . By adopting this B * Kane , the highest zT of 1.54 and 0.27 are predicted in (Bi,Sb) 2 Te 3 and Ta 4 SiTe 4 , which could be achieved by further optimizing the η and ξ . Understanding low lattice thermal conductivity Lattice thermal conductivities, κ L of Pb 7 Bi 4 Se 13 samples are presented in Fig. 5a . The κ L is estimated by subtracting electronic thermal conductivity, κ e from total thermal conductivity. The κ e is estimated by using the Wiedemann–Franz equation, κ e = LσT . The κ L ranges from 0.44 to 0.29 Wm −1 K −1 at 300 K, and decreases with rising temperature. This decline deviates from the T −1 tendency dominated by Umklapp phonon-phonon scattering, which implies strong defect-phonon scattering. Specifically, the κ L for Pb 7 Bi 4 Se 13 with n H of 1.2 × 10 20 cm −3 decreases from 0.33 Wm −1 K −1 at 300 K to 0.17 Wm −1 K −1 at 800 K. This low κ L is comparable to that of state-of-the-art TE materials, such as 0.18 Wm −1 K −1 for CsAg 5 Te 3 [44] , 0.13 Wm −1 K −1 for both (Ge,Mn,Sb)Te [45] and Bi 1− x Pb x CuSeO [46] . To further assess the intrinsic Umklapp phonon interaction, sound speeds were measured. The related physical parameters were calculated and tabulated in Table S6 . The mean sound speed for Pb 7 Bi 4 Se 13 is as low as 1553 ms −1 , and the Grüneisen parameter γ G is 2.2. This large γ G is indicative of soft chemical bonding and strong lattice vibration anharmonicity, which is comparable with γ G of 2.6 for Ag 9 GaSe 6 [19] , 2.1 for AgSbTe 2 [47] , 1.7 for K 2 Bi 8 Se 13 [48] , 1.7 for BiSe [49] , and 1.6 for Cu 17.6 Fe 17.6 Se 32 [50] , etc. The calculated Debye temperature ( Θ D ) is as low as 148 K, comparable to 147 K in Ag 9 GaSe 6 with liquid-like thermal conductivity [33] . The large Grüneisen parameter and low Debye temperature lead to large lattice anharmonicity and strong Umklapp phonon–phonon scattering. Fig. 5: Lattice thermal conductivity and phonon-related calculations. a Lattice thermal conductivity, κ L . b T dependence of C p / T 3 . The circle is the experimental data and the line is established by using a Debye and three Einstein modes. c Phonon dispersions and atom-projected phonon DOS of the low-frequency phonons up to f = 1.0 THz. Transverse acoustic phonons, TA1 and TA2 are plotted in red and orange colors. Longitudinal acoustic phonon, LA, is in the blue line. Optical phonons are in black lines. In the low-frequency region, the dominant contribution stems from Pb atoms. d Grüneisen dispersions. Displacement patterns of e the low-frequency optical phonon at Γ point, and f low-frequency TA1 mode at Γ point. Full size image The low-temperature heat capacity in Fig. S 13 shows the non-linear relationship of C p / T vs. T 2 . This inconsistency with the conventional Debye model implies the existence of localized Einstein oscillator modes. A broad maximum appears around 8 K in the T dependence of C p / T 3 (Fig. 5b ). This additional contribution to heat capacity is a signature of localized optical phonon modes, frequently found in TEs with low thermal conductivities [17] , [51] . To quantitatively describe the heat capacity, a combined Debye–Einstein model is adopted (see Table S7 ). Three low-frequency Einstein vibration modes are utilized for a full description of the measured data. And the Einstein characteristic temperatures are Θ E 1 = 13 K, Θ E 2 = 33 K, and Θ E 3 = 119 K, respectively. To understand the origin of low thermal conductivity, first-principles phonon calculations were performed to study lattice dynamics. Phonon dispersions and atom projected phonon DOS in the low-frequency region are presented in Fig. 5c . The full phonon spectrum and DOS is demonstrated in Fig. S 14 . Intriguingly, optical phonon modes with low energies at Γ point can be observed around 0.28, 0.45, and 0.59 THz, respectively. These lowest optical phonons are in good agreement with experimentally verified lowest Einstein modes observed in Fig. 5b . Actually, the low-energy vibrational modes in phonon DOS have been directly observed in (PbSe) 5 (Bi 2 Se 3 ) 3m by the inelastic neutron scattering measurement [52] , which shares similar structural complexity and compositions with Pb 7 Bi 4 Se 13 . Besides, the maxima centered below 10 K in the relationship of T ~ C p / T 3 have also been observed in (PbSe) 5 (Bi 2 Se 3 ) 3m . These features have also been reported in compounds with low thermal conductivities, such as BaGa 5 and InTe [53] , [54] . The low-lying optical phonons couple with heat-carrying acoustic phonons, decreasing group velocities and thereby restraining heat transport. Similar low-frequency optical phonons have been observed in typical TE materials with usually low κ L , such as MgAgSb [20] , TIInTe 2 [51] , and AgBi 3 S 5 [18] . Atom-projected phonon DOS shows the dominant contribution from Pb atoms in the low-frequency region (<1.0 THz), strongly correlated to its 6 s 2 lone pair electrons [31] , [55] . The specific vibration pattern of this lowest optical phonon at Γ point is visualized in Fig. 5e . According to κ L ~ γ G −2 , γ G is a measure of anharmonicity of phonon modes and is inversely proportional to lattice thermal conductivity. To quantitively evaluate lattice anharmonicity, we plot the Grüneisen dispersions of acoustic phonons in Fig. 5d . A striking feature is the anomaly large values of γ G on A-Γ, Y 2 -Γ, and M 2 -Γ paths, indicating largely enhanced anharmonicity. Specifically, the γ G of TA1 at Γ point reaches up to a high value of 16. Such high γ G indeed demonstrates strong anharmonicity and intensified the Umklapp phonon-phonon scattering. And this specific vibration pattern is depicted in Fig. 5f . We further used the quasi-harmonic approximation methods to calculate the mode-averaged γ G to be 2.0, in good agreement with the experimental γ G of 2.2. Therefore, the low thermal conductivity has an intimate relationship with localized low-frequency optical phonon modes and the large anharmonicity of acoustic phonons. The SOC effect on phonon calculation has also been considered, which demonstrates a limited effect on the calculated phonon spectra (see Fig. S 14 ). Coexistence of diverse defects Nanoscale defects also play a significant role in the low thermal conductivity. To elucidate defect-phonon scattering sources, a microstructural investigation by using a spherical aberration-corrected scanning transmission electron microscope (Cs-corrected STEM) was employed on Pb 7 Bi 4 Se 13 with n H of 1.2 × 10 20 cm −3 . High-angle annular dark-field (HAADF)-STEM images in Fig. 6a, b clearly show the periodic defective stripes, with a length beyond 30 nm and a width of ~3 nm, embedded in the host matrix of Pb 7 Bi 4 Se 13 . The defective stripes include high-density of stacking faults, shown by the white arrows in Fig. 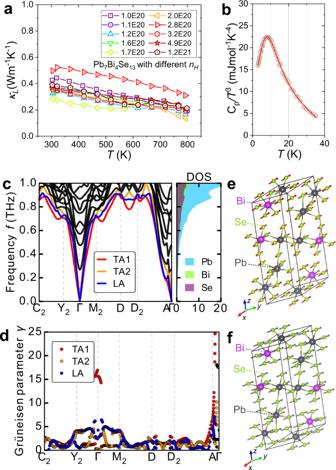Fig. 5: Lattice thermal conductivity and phonon-related calculations. aLattice thermal conductivity, κL.bTdependence ofCp/T3. The circle is the experimental data and the line is established by using a Debye and three Einstein modes.cPhonon dispersions and atom-projected phonon DOS of the low-frequency phonons up tof= 1.0 THz. Transverse acoustic phonons, TA1 and TA2 are plotted in red and orange colors. Longitudinal acoustic phonon, LA, is in the blue line. Optical phonons are in black lines. In the low-frequency region, the dominant contribution stems from Pb atoms.dGrüneisen dispersions. Displacement patterns ofethe low-frequency optical phonon at Γ point, andflow-frequency TA1 mode at Γ point. 6b . The elemental mapping in Fig. S 15 verifies the homogeneously distributed elements along with defective stripes. The strain map profiles ( ε xx ) in Fig. 6a1, b1 are derived by geometric phase analysis (GPA), which semi-quantitatively evaluate spatially distributed strain fields. Intriguingly, the periodic strain lines are captured (labeled by black arrows) and demonstrate the intense strains along with these defective stripes in Fig. 6a, b . The strain analysis of ε yy is presented in Fig. S 15 . In addition, dislocation cores are also observed, highlighted by white circles. 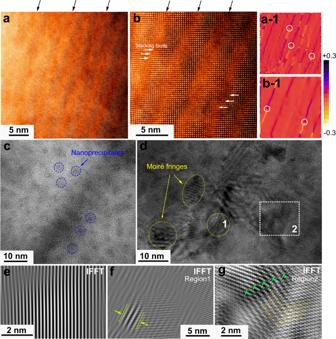Fig. 6: Nanoscale defects. a,bHAADF-STEM images showing periodic defective stripes, marked by black arrows. High-density stacking faults are observed and indicated by white arrows.a-1,b-1Corresponding GPA results (εxx) of (a) and (b), revealing intense lattice strains. The periodic strain lines are indicated by black arrows, in which dislocation cores are marked by white circles.cHRTEM image showing the high number density of nanoscale precipitates, encircled by blue dotted lines.dTEM image demonstrating strong moiré fringes indicated by yellow ellipses and highly distorted lattice marked by a white square. Inverse fast Fourier transform (IFFT) images of selected regions.eDefect-rare region,fdefect-rich region 1, full of moiré fringes, andgregion 2, filled up with dislocation arrays and twinned grain boundaries. Figure 6c presents the irregularly shaped nanoscale precipitates embedded in the host matrix, marked by the blue dotted circles. These high number density of nanoscale precipitates demonstrates the size of several nanometers. Diverse lattice imperfections have been evidently observed in Fig. 6d . The moiré fringes, marked by the yellow ellipses, distribute around the dark-contrast precipitates. These strong moiré fringes originate from the interference between different sets of lattice planes, indicating local mass and strain fluctuations. Figure 6e shows the enlarged region from the inverse fast Fourier transform of Fig. S 16c . In sharp contrast to the slightly distorted lattice in Fig. 6e , another two regions in Fig. 6f, g highlight the crystal imperfections. In Fig. 6f , moiré patterns are highlighted by the pleated structure, marked by the yellow lines. In Fig. 6g , the coexistence of dislocation arrays and nanoscale twined structures, demonstrated by green symbols and parallel brown lines, respectively. Numerous nano-precipitates and dislocations can also be observed in Fig. S 16 . The coexistence of periodic defective stripes, nanoprecipitates, dislocation, and Moiré fringes play a significant role in scattering phonon with different length scales, which strongly suppresses lattice thermal conductivity. Fig. 6: Nanoscale defects. a , b HAADF-STEM images showing periodic defective stripes, marked by black arrows. High-density stacking faults are observed and indicated by white arrows. a-1 , b-1 Corresponding GPA results (ε xx ) of ( a ) and ( b ), revealing intense lattice strains. The periodic strain lines are indicated by black arrows, in which dislocation cores are marked by white circles. c HRTEM image showing the high number density of nanoscale precipitates, encircled by blue dotted lines. d TEM image demonstrating strong moiré fringes indicated by yellow ellipses and highly distorted lattice marked by a white square. Inverse fast Fourier transform (IFFT) images of selected regions. e Defect-rare region, f defect-rich region 1, full of moiré fringes, and g region 2, filled up with dislocation arrays and twinned grain boundaries. Full size image In this work, we report the discovery of a unique TE material, Pb 7 Bi 4 Se 13 based lillianites. A high peak zT of 1.35 at 800 K and a decent average zT of 0.92 from 450 to 800 K are achieved for n -type (Pb 0.95 Ga 0.05 )Bi 4 Se 13 . This is the highest TE performance realized in lillianites. For Pb 7 Bi 4 Se 13 , conduction bands are highly nested at Y 2 and M 2 points. Besides, these nested conduction bands at Y 2 and M 2 also share similar energies, demonstrating a strong signature of band convergence. The synergistic effect of band nestification and convergence leads to higher band degeneracy and superior electrical properties. It provides an alternative approach to improve valley degeneracy for low-symmetry TE systems. These electronic band features are rarely documented in compounds with lower crystal symmetries and are comparable to typical n -type TE materials, such as PbTe and CoSb 3 , which both demonstrate multiple degenerated bands as well as narrow-band gaps ( E g = ~0.3 eV for PbTe and ~0.23 eV for CoSb 3 ) [7] , [8] . For PbTe, conduction bands consist of one Kane band at the L point. The full valley degeneracy, N v for L are 4. For CoSb 3 , conduction bands are composed of one Kane band at Γ point ( N v = 3) and one parabolic band along the Γ–N line ( N v = 12). The conventional quality factor neglects the features of band nonparabolicity and bandgap, whose application is severely limited in narrow-gap TE materials. A unique quality factor, B * Kane is deliberately established here, which can break previous limitations and provide an effective method to predict and evaluate TE properties. Furthermore, a low lattice thermal conductivity, 0.17 Wm −1 K −1 is achieved at 800 K. The intrinsic and extrinsic phonon scattering sources synergistically suppress phonon transport and achieve the ultralow lattice thermal conductivity. The intrinsic component stems from strong anharmonicity of an acoustic phonon with large Grüneisen parameter ( γ G = 16), localized low-frequency optical phonons (<0.6 THz), and low Debye temperature ( Θ D = 148 K). Moreover, the extrinsic nanoscale lattice imperfections, including periodic defective stripes, nano-precipitates, dislocations, and Moiré fringes, facilitate to impede heat transport. This work could rekindle the hope and vision of lillianites as promising high-performance TE materials. Furthermore, the unique quality factor paves an attractive route to accelerate the exploration for TE compounds with resembling band characteristics. Synthesis Pb shots (99.99%), Ag shots (99.999%), Ga chunks (99.999%), In shots (99.999%), Se shots (99.999%), and I pieces (99.999%) were purchased from Sigma-Aldrich. Firstly, precursors of Pb 1− x M x Se (M = Ga, In or Ag), PbSe 1− x I x , and Bi 2 Se 3 were prepared by loading the raw materials into vacuum quartz tubes according to the stoichiometric ratio, then heated up to 1373 K for 24 h in a box furnace. Ingots of (Pb 1− x Ga x ) 7 Bi 4 Se 13 , (Pb 1− x In x ) 7 Bi 4 Se 13 , (Pb 1− x Ag x ) 7 Bi 4 Se 13 and Pb 7 Bi 4 Se 13− x I x were prepared by loading precursors Pb 1− x M x Se ( M = Ga, In or Ag) or PbSe 1− x I x and Bi 2 Se 3 into ball-milling vials in a glove box (O 2 and H 2 O content < 0.1 ppm), according to the normal compositions. Precursors were mechanically alloyed by high-energy ball-milling (SPEX 8000D). To ensure full and homogeneous milling, the chemicals attached to the inner wall of vials were scratched out in the glove box after ball-milling for 1.5 h. This process was repeated eight times. After the long-term ball-milling, the powders were pressed into pellets in the glove box. The pellets were subsequently flame-sealed into vacuum quartz tubes. Then, the quartz tubes were transferred into a box furnace and heated to 573 K in 24 h, dwelled for 72 h, followed by heating up to 850 K in 24 h, and then soaked for two weeks. Subsequently, they were cooled down to room temperature in 12 h. These ingots were crushed into powders by mortar and pestle in a glove box and densified by an SPS system (Ed-PasIVJ, 6T-3P-30, Japan) at 823 K for 10 min with an axial pressure of 75 MPa under vacuum. The sintered pellets were then cut into a 3 × 3 × 12 mm 3 rectangular bar and into a ∅ 12.7 × 2 mm disk for measurements. Characterization Laboratory X-ray patterns were collected on PANalytical X’pert Pro powder diffractometer with Cu target (operating under 40 kV and 30 mA). The electrical conductivity and Seebeck coefficient were measured simultaneously using ZEM-3 system (ULVAC-RIKO, Japan). The thermal conductivity was calculated by κ = DC p ρ , in which the Dulong–Petit specific heat was taken as the specific heat ( C p ), the pellet density ( ρ ) was calculated by the geometrical method and the thermal diffusivity ( D ) was measured using the lasher flash method (DLF 1200, TA Instruments, USA). Room temperature charge carrier concentration was determined from the Hall coefficient measurement using the Van der Pauw method (Bio-Rad Microscience, Hall measurement system HL5500, USA). High-temperature carrier concentration, Hall coefficient and Hall mobility were collected at the homemade device with the Van der Pauw method. Cross-sectional transmission electron microscopy (TEM) samples were prepared using the conventional in situ lift-out method, which was performed on a dual-beam scanning electron microscope-focused ion beam (SEM-FIB) instrument (Crossbeam XB540, Zeiss, Germany) with an attached micromanipulator (OmniProbe 400, Oxford Instrument, UK). High-angle annular dark-field scanning transmission electron microscopy (HAADF-STEM) images were taken in an aberration-correlated JEOL ARM-200F operating at 200 kV. The collection angle of the HAADF-STEM image was from 80 to 250 mrad. EDS mapping was carried out by an Oxford X-Max EDS detector. The microstructures were characterized by a field-emission gun transmission electron microscope (FEG-TEM, JEM-2100F, JEOL, Japan). TEM and HRTEM images were taken using a Gatan Ultrascan 1000XP CCD. The samples for the compressive test, with a size of ∅ 2 × 4 mm, were machined using an electron discharge machining machine, conducted by an Instron 3384 Electromechanical Universal Testing Machines. The nanoindentation investigation was performed on Hysitron TI-980 Triboindenter nanoindenter (Bruker Nano Surfaces, USA). Electronic structure and phonon calculations First-principles density functional theory (DFT) calculations were performed using the Vienna Ab-initio Simulation Package [56] , [57] . The generalized gradient approximation in the Perdew–Burke–Ernzerhof parametrization [58] was used as the exchange-correlation functional. The cutoff energy was set to 400 eV which has been sufficient to guarantee accuracy. We used a primitive cell of Pb 7 Bi 4 Se 13 including 24 atoms in modeling the electronic properties. The energy convergency threshold and force convergency threshold in the structural optimization were 10 −8 eV and 10 −4 eV Å −1 , respectively. A k -mesh of 9 × 9 × 3 was used to sample the k points in the Brillouin zone. The rigid band approximation was used to model the n -type and p -type Pb 7 Bi 4 Se 13 . Specifically, the electron/hole doping in Pb 7 Bi 4 Se 13 is achieved by adding extra electrons/holes to the system with the same amount of uniform positive/negative charge in the background. Within the framework of rigid band approximation, we find the overall shape of band structures are almost unchanged except the Fermi level shift, hence we only show the calculated Fermi level of 0.05 electron- and hole-doped Pb 7 Bi 4 Se 13 in Fig. 2a of the main text. The corresponding Fermi surfaces were calculated by using a very dense 45 × 45 × 15 k -mesh to ensure the accuracy of calculations for metallic states. To evaluate the lattice dynamic properties, we used the finite displacement supercell method to calculate the phonon spectrum and phonon density of states and used the quasi-harmonic method to calculate the Grüneisen parameter. Both the finite displacement supercell method and quasi-harmonic method implemented in Phonopy [59] were used. In addition, the finite displacement supercell method was used with the 3 × 3 × 1 supercell (216 atoms) of the primitive cell with a finite displacement of 0.1 Å. The crystal structures and displacement patterns were all visualized using VESTA software [60] . When computing the phonon density of states of mode-averaged Grüneisen, we used a q -mesh of 20 × 20 × 20.